CEP63 deficiency promotes p53-dependent microcephaly and reveals a role for the centrosome in meiotic recombination CEP63 is a centrosomal protein that facilitates centriole duplication and is regulated by the DNA damage response. Mutations in CEP63 cause Seckel syndrome, a human disease characterized by microcephaly and dwarfism. Here we demonstrate that Cep63 -deficient mice recapitulate Seckel syndrome pathology. The attrition of neural progenitor cells involves p53-dependent cell death, and brain size is rescued by the deletion of p53. Cell death is not the result of an aberrant DNA damage response but is triggered by centrosome-based mitotic errors. In addition, Cep63 loss severely impairs meiotic recombination, leading to profound male infertility. Cep63 -deficient spermatocytes display numerical and structural centrosome aberrations, chromosome entanglements and defective telomere clustering, suggesting that a reduction in centrosome-mediated chromosome movements underlies recombination failure. Our results provide novel insight into the molecular pathology of microcephaly and establish a role for the centrosome in meiotic recombination. Many mutations in genes encoding proteins involved in the DNA damage response (DDR) and/or centrosomal functions have been identified in human patients with autosomal recessive primary microcephaly (MCPH) or Seckel syndrome (MCPH accompanied by dwarfism) [1] , [2] , [3] , [4] , [5] , [6] , [7] , [8] , [9] , [10] , [11] , [12] , [13] . This has suggested that crosstalk between the DDR and the centrosome may be highly relevant to the aetiology of microcephaly. Supporting this idea, several MCPH/Seckel proteins, such as MCPH1 and CEP152, have been implicated in both centrosomal and DDR functions [9] , [14] , [15] , [16] . In addition, signalling through the central transducer of DNA damage, ATR (also mutated in Seckel syndrome), involves the PCNT (pericentrin)/MCPH1-dependent localization of CHK1 to the centrosome [17] , [18] . The development of microcephaly has been attributed to the attrition of neural progenitor cells (NPCs) due to defective self-renewal capacity or as a result of sporadic DNA damage, resulting from checkpoint defects, DNA repair deficiencies, replication stress, mitotic errors and increased apoptosis [4] , [19] . In addition, defective nuclear partitioning and the death of migrating differentiated cells have also been shown to influence cortical development [20] . The relative importance of these, or other mechanisms, in the pathology of microcephaly in MCPH and Seckel syndrome and to what extent other organ systems are affected remain open questions. The centrosomal protein CEP63 was identified as a target of the apical DDR kinases ATM and ATR in mitosis and was recently shown to promote efficient centriole duplication through interactions with CEP152, which has also been implicated in ATM signalling [5] , [9] , [21] , [22] . Both CEP63 and CEP152 mutations have been identified in Seckel syndrome and additional CEP152 mutations underlie MCPH [5] , [7] , [9] . Here we describe the phenotypic analysis of mice lacking expression of the Cep63 gene. These animals recapitulate the pathological outcomes reported in human patients with CEP63 mutations, including growth defects and microcephaly [5] . Brain development in Cep63 mutants is impaired by increased cell death and reduced numbers of NPCs, which can be rescued by the deletion of p53, but not the ATM or CHK2 kinases. Cep63 -deficient cells and tissues do not show obvious defects in DNA damage signalling, but exhibit impaired centriole duplication accompanied by defects in bipolar spindle assembly and function. In addition, we find that male Cep63 -deficient mice are infertile, exhibiting severe defects in meiotic recombination and a complete block in the generation of mature sperm. We show that in spermatocytes, centrosome duplication is coordinated with the progression of meiotic prophase. In Cep63 -deficient males, centrosomes fail to duplicate and display compromised structural integrity, and chromosome dynamics are impaired. Collectively, our results shed light on the complex aetiology of microcephaly and reveal a novel and essential role for centrosomes in promoting recombination during mammalian meiosis. Cep63 deficiency leads to growth defects and microcephaly Previous work demonstrated an interaction between CEP63 and CEP152, two proteins encoded by established MCPH and Seckel syndrome genes [5] , [9] , [22] , [23] . To determine whether Cep63 deficiency in mice would phenocopy the human diseases, we generated animals with a gene-trapped allele of the Cep63 gene ( Cep63 T ; ref. 22 ). Cep63 T/T pups were born at expected Mendelian ratios and newborn animals were similar in weight to wild type (WT) or heterozygous littermates ( Fig. 1a ). However, by 1–2 months, Cep63 T/T mice exhibited a significant reduction in the average weight ( Fig. 1b,c ), indicating growth retardation, a hallmark of human Seckel syndrome patients [3] , [5] , [9] . 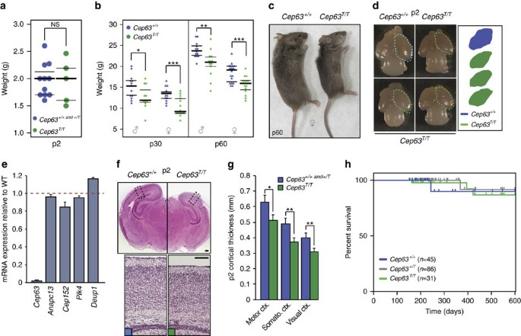Figure 1: Cep63 deficiency leads to growth defects and microcephaly. (a) Weights of newborn mice (p2) of the indicated genotype (Cep63+/+, +/Tn=11,Cep63T/Tn=5 pups). (b) Weight of p30 and p60 mice of the indicated sex and genotype (n=13, 11, 16, 14, 13, 13, 18 and 14 animals, respectively). (c) Examples of female littermateCep63+/+andCep63T/Tmice at p60. (d) Examples of p2-dissected brains of the indicated genotype with the relative cerebral cortex area compared. (e) Quantitative real-time PCR of the indicated genes using cDNA prepared from the cortex of p2 animals. Levels of mRNA expression relative to WT littermates is graphed usingB2MandACTBas a reference. (n=3 animals per genotype). (f) Haematoxylin and eosin (H&E)-stained coronal sections ofCep63+/+andCep63T/Tcortices from p2 animals with approximate area of higher magnification indicated (top panels). Higher-magnification panels of the motor cortex stained with H&E (bottom panels, scale bars, 0.2 mm). (g) Quantification of p2 cortical thickness from the indicated genotypes and area (two hemispheres per brain section were averaged,n=3 animals is graphed). (h) Kaplan–Meier curve of mouse survival. No significant differences (log-rank test) were observed over 600 days. The number of animals per genotype is indicated. Ina,b, the median (thick line) with the first and third quartiles of the box plot (thin lines) are indicated. Ine,g,graphics with error bars represent the average plus s.d. Asterisks denote statistical significance (NS, not significant, *Pvalue <0.05, **Pvalue <0.01 and ***Pvalue <0.001) determined by the unpaired two-way Student’st-test (a,g) or the unpaired two-way Wilcoxon rank-sum test (b). Figure 1: Cep63 deficiency leads to growth defects and microcephaly. ( a ) Weights of newborn mice (p2) of the indicated genotype ( Cep63 +/+, +/T n =11, Cep63 T/T n =5 pups). ( b ) Weight of p30 and p60 mice of the indicated sex and genotype ( n =13, 11, 16, 14, 13, 13, 18 and 14 animals, respectively). ( c ) Examples of female littermate Cep63 +/+ and Cep63 T/T mice at p60. ( d ) Examples of p2-dissected brains of the indicated genotype with the relative cerebral cortex area compared. ( e ) Quantitative real-time PCR of the indicated genes using cDNA prepared from the cortex of p2 animals. Levels of mRNA expression relative to WT littermates is graphed using B2M and ACTB as a reference. ( n =3 animals per genotype). ( f ) Haematoxylin and eosin (H&E)-stained coronal sections of Cep63 +/+ and Cep63 T/T cortices from p2 animals with approximate area of higher magnification indicated (top panels). Higher-magnification panels of the motor cortex stained with H&E (bottom panels, scale bars, 0.2 mm). ( g ) Quantification of p2 cortical thickness from the indicated genotypes and area (two hemispheres per brain section were averaged, n =3 animals is graphed). ( h ) Kaplan–Meier curve of mouse survival. No significant differences (log-rank test) were observed over 600 days. The number of animals per genotype is indicated. In a , b , the median (thick line) with the first and third quartiles of the box plot (thin lines) are indicated. In e , g, graphics with error bars represent the average plus s.d. Asterisks denote statistical significance (NS, not significant, * P value <0.05, ** P value <0.01 and *** P value <0.001) determined by the unpaired two-way Student’s t -test ( a , g ) or the unpaired two-way Wilcoxon rank-sum test ( b ). Full size image As CEP63 mutations cause microcephaly in humans [5] , we examined neurodevelopment in Cep63 T/T animals. In newborn (p2) animals, forebrain size was reduced compared with WT, despite similar body weight ( Fig. 1a,d ). Strongly reduced Cep63 mRNA levels were confirmed in the cortex of Cep63 T/T mice ( Fig. 1e ), whereas Anapc13 , a gene positioned head-to-head with Cep63 , was not affected. In addition, we did not observe changes in the expression of key centriole duplication components Plk4 and Cep152 , or the Cep63 paralogue, Deup1 ( Fig. 1e ). Characteristic of MCPH and Seckel syndrome, cortical development was impaired ( Fig. 1f ) and examination of p2 cortices revealed a consistent reduction in thickness at all positions examined ( Fig. 1g ). Despite reduced cortex size, longevity of Cep63 T/T animals was similar to WT and no obvious motor defects were observed in an aging cohort ( Fig. 1h ). Together, these data demonstrated that Cep63 deficiency recapitulated the major pathologies of Seckel syndrome. Mitotic defects and cell death in neural progenitors The attrition of NPCs in the cortex has been clearly linked to microcephaly, and can be provoked by increased DNA damage, impaired NPC self-renewal or centrosomal defects [24] , [25] , [26] , [27] . CEP63 has been linked to the DDR and its deficiency leads to centriole loss due to impaired recruitment of CEP152 (refs 5 , 22 ). We therefore examined colocalization of CEP152 or CEP63 with the centrosome marker γ-tubulin in the developing cortex of E14.5 embryos [5] , [22] . While focal CEP152 was readily detected at centrosomes in WT animals, we could not identify focal staining that overlapped with γ-tubulin in Cep63 T/T mice ( Fig. 2a ). Since Cep152 mRNA expression levels in the Cep63 T/T brain were not reduced relative to WT ( Fig. 1e ) and similar amounts of CEP152 protein could be immunoprecipitated from WT and Cep63 T/T tissues ( Supplementary Fig. 1 ), this likely reflects a defect in the centrosomal recruitment of CEP152, similar to what we have previously reported in Cep63 T/T mouse embryonic fibroblasts (MEFs) [22] . In addition, while we could readily detect CEP63 localization to the centrosomes in WT E14.5 embryos, we did not observe its localization in Cep63 T/T embryos, consistent with its reduced levels of expression ( Figs 1e and 2b , and Supplementary Fig. 1 ). 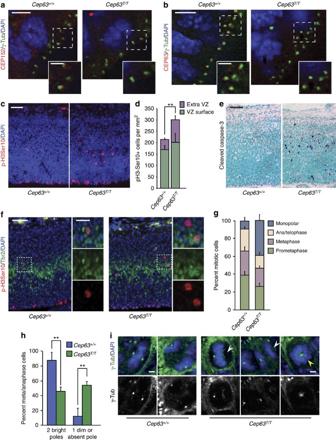Figure 2: Impaired CEP152 localization and mitotic defects inCep63-deficient brains. (a) CEP152 is detectable at centrosomes, marked by γ-tubulin (γ-Tub), in the cortex of WT (left panel) but notCep63T/T(right panel) E14.5 embryos. (scale bars, 5 μm (left) and 2 μm (right)). (b) CEP63 is detectable at centrosomes, marked by γ−tubulin, in the cortex of WT (left panel) but notCep63T/TE14.5 embryos (right panel). (scale bars, 5 μm (left) and 2 μm (right)). (c) Increased number and defective localization of mitotic cells (positive for p-H3Ser10) in the E14.5 cortex ofCep63T/Tembryos (right panel) compared with WT (left panel). (scale bar, 50 μm). (d) Quantification of VZ surface and extra-VZ p-H3Ser10-positive mitoses in the indicated genotype (n=5 and 3 animals per genotype, respectively). (e) Increased cleaved caspase-3 staining indicates increased cell death in the cortex ofCep63T/Tembryos at E14.5 (right panel) compared with WT (left panel). (scale bar, 50 μm). (f) Some misplaced mitotic cells in theCep63T/Tcortex are intermediate progenitors identified by positivity for Tbr2. (scale bars, 50 μm (left) and 20 μm (right)). (g) Scoring of mitotic configurations in the E14.5 VZ. Categories and genotypes are indicated (n=3 animals per genotype used, 102Cep63+/+and 150Cep63T/Tcells scored). (h) Scoring of γ-tubulin foci in metaphase and anaphase cells in VZ of E14.5 brain cortex. Mitotic cells were identified by staining sections with DAPI (DNA) and γ-tubulin (centrosome), and scored by morphology and γ-tubulin spot numbers (n=3 animals per genotype used, 64Cep63+/+and 62Cep63T/Tcells scored). (i) Example images of acentrosomal (white arrowheads) and monopolar (yellow arrowhead) mitoses inCep63T/Tembryos (scale bar, 2 μm). All graphics with error bars are presented as the average plus s.d. Asterisks denote statistical significance (**Pvalue <0.01) determined by the unpaired two-way Student’st-test (d,h). Figure 2: Impaired CEP152 localization and mitotic defects in Cep63 -deficient brains. ( a ) CEP152 is detectable at centrosomes, marked by γ-tubulin (γ-Tub), in the cortex of WT (left panel) but not Cep63 T/T (right panel) E14.5 embryos. (scale bars, 5 μm (left) and 2 μm (right)). ( b ) CEP63 is detectable at centrosomes, marked by γ−tubulin, in the cortex of WT (left panel) but not Cep63 T/T E14.5 embryos (right panel). (scale bars, 5 μm (left) and 2 μm (right)). ( c ) Increased number and defective localization of mitotic cells (positive for p-H3Ser10) in the E14.5 cortex of Cep63 T/T embryos (right panel) compared with WT (left panel). (scale bar, 50 μm). ( d ) Quantification of VZ surface and extra-VZ p-H3Ser10-positive mitoses in the indicated genotype ( n =5 and 3 animals per genotype, respectively). ( e ) Increased cleaved caspase-3 staining indicates increased cell death in the cortex of Cep63 T/T embryos at E14.5 (right panel) compared with WT (left panel). (scale bar, 50 μm). ( f ) Some misplaced mitotic cells in the Cep63 T/T cortex are intermediate progenitors identified by positivity for Tbr2. (scale bars, 50 μm (left) and 20 μm (right)). ( g ) Scoring of mitotic configurations in the E14.5 VZ. Categories and genotypes are indicated ( n =3 animals per genotype used, 102 Cep63 +/+ and 150 Cep63 T/T cells scored). ( h ) Scoring of γ-tubulin foci in metaphase and anaphase cells in VZ of E14.5 brain cortex. Mitotic cells were identified by staining sections with DAPI (DNA) and γ-tubulin (centrosome), and scored by morphology and γ-tubulin spot numbers ( n =3 animals per genotype used, 64 Cep63 +/+ and 62 Cep63 T/T cells scored). ( i ) Example images of acentrosomal (white arrowheads) and monopolar (yellow arrowhead) mitoses in Cep63 T/T embryos (scale bar, 2 μm). All graphics with error bars are presented as the average plus s.d. Asterisks denote statistical significance (** P value <0.01) determined by the unpaired two-way Student’s t -test ( d , h ). Full size image As defective CEP63/CEP152 recruitment and impaired centriole duplication could lead to mitotic defects, we next examined the status of the proliferative NPC population and cell death in the developing cortex of E14.5 animals using antibodies against histone H3 phosphorylated on serine10 (p-H3Ser10), a marker of mitosis, and the apoptotic marker cleaved caspase-3. At E14.5, we observed slightly elevated numbers of p-H3Ser10-positive cells in the ventricular zone (VZ) of the cortex of Cep63 T/T animals compared with WT ( Fig. 2c,d ) and highly elevated levels of cleaved caspase-3 throughout the cortex ( Fig. 2e ). In addition, we observed an increased number of extra-VZ p-H3Ser10-positive cells, similar to what has been recently reported in mice lacking SAS4 ( Fig. 2c,d ) [25] . We examined the identities of these misplaced proliferating cells using a marker for intermediate progenitors, Tbr2, and found that this displaced population was composed of both Tbr2-positive and -negative cells, suggesting that it is composed of multiple classes of NPCs, including radial glial progenitors and intermediate progenitors ( Fig. 2f ). The increased number of mitotic cells, coupled with the increased cell death we observed, suggested the presence of mitotic errors or delays. We next examined the spindle configurations in WT and Cep63 T/T cortices using anti-γ-tubulin antibodies and 4,6-diamidino-2-phenylindole (DAPI) to label centrosomes and DNA, respectively. This revealed a strong increase in the percentage of monopolar spindle configurations in the VZ of Cep63 T/T cortices ( Fig. 2g ). Moreover, in cells with bipolar spindles, the γ-tubulin signal at one of the poles was frequently dim or absent, suggesting that spindle poles were formed by defective centrosomes or were acentrosomal ( Fig. 2h,i ). Collectively, these data indicated that CEP63 ensures proper duplication and formation of functional centrosomes, which in NPCs is crucial for mitotic fidelity, proper positioning of proliferating NPCs and cell survival. CEP63 deficiency leads to p53-dependent NPC attrition NPCs lacking centrioles are misplaced from the subventricular zone (SVZ), exhibit prolonged mitoses and trigger cell death through p53 signalling [26] , [28] , [29] . However, opposing genetic interactions with p53 deficiency have been described in other models of microcephaly, such as in Atr -deficient mice, and CEP63 has been previously linked to the ATM/ATR-dependent DDR [24] , [28] , [30] , [31] . To address the cell death pathways triggered by loss of CEP63, we stained the cortices of E14.5 mice with antibodies for the DNA break marker γH2AX or p53. Little staining for either marker was observed in WT animals while a striking upregulation of p53 was apparent in the cortex of Cep63 T/T embryos ( Fig. 3a–d ). The majority of p53 staining was observed in the proliferating cell nuclear antigen (PCNA)-positive cells of the VZ, suggesting that p53 is primarily activated in the proliferating NPC population ( Fig. 3b ). Only a minor increase in γH2AX was seen in the cortex of Cep63 T/T animals but the staining was not punctate, as expected for DNA breaks, and may reflect cells already undergoing apoptosis ( Fig. 3c,d ). 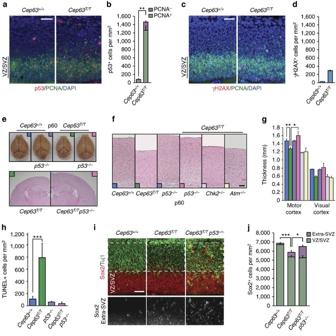Figure 3: p53-dependent attrition of neural progenitors inCep63-deficient embryos. (a) Strong induction of p53 in the cortex ofCep63T/Tembryos compared with WT at E14.5 (scale bar, 50 μm). (b) Scoring of p53-positive cells ina(n=2 animals per genotype). (c) Slightly increased levels of γH2AX can be visualized in the E14.5 cortex ofCep63T/Tembryos compared with WT (scale bar, 50 μm). (d) Quantification of γH2AX-positive cells inc(n=1 animal per genotype). (e) Dissected p60 brains (upper panel) and representative coronal sections fromCep63T/TandCep63T/Tp53−/−mice (lower panel). (f) Representative examples illustrating relative p60 motor cortex thickness in mice of the indicated genotype (scale bar, 0.2 mm). (g) Measurement of cortex thickness from sections of the motor or visual cortex with colours corresponding to genotypes inf(n=3, 3, 2, 3, 2 and 2 animals used per genotype, respectively). (h) Quantification of TUNEL staining (n=6, 10, 4 and 4 sections per animal were scored, sections from 2, 3, 1 and 1 animals per genotype were used, respectively). (i) Misplacement of neural/stem cell progenitors (Sox2 positive) inCep63T/TandCep63T/Tp53−/−animals (scale bar, 50 μm). (j) Rescue of misplaced progenitors inCep63T/Tp53−/−animals compared withCep63T/T(n=5, 3 and 3 animals per genotype, respectively). All graphics with error bars are presented as the average plus s.d. Asterisks denote statistical significance (*Pvalue <0.05, **Pvalue <0.01 and ***Pvalue<0.001) determined by the unpaired two-way Student’st-test (b,g,h,j). Figure 3: p53-dependent attrition of neural progenitors in Cep63 -deficient embryos. ( a ) Strong induction of p53 in the cortex of Cep63 T/T embryos compared with WT at E14.5 (scale bar, 50 μm). ( b ) Scoring of p53-positive cells in a ( n =2 animals per genotype). ( c ) Slightly increased levels of γH2AX can be visualized in the E14.5 cortex of Cep63 T/T embryos compared with WT (scale bar, 50 μm). ( d ) Quantification of γH2AX-positive cells in c ( n =1 animal per genotype). ( e ) Dissected p60 brains (upper panel) and representative coronal sections from Cep63 T/T and Cep63 T/T p53 −/− mice (lower panel). ( f ) Representative examples illustrating relative p60 motor cortex thickness in mice of the indicated genotype (scale bar, 0.2 mm). ( g ) Measurement of cortex thickness from sections of the motor or visual cortex with colours corresponding to genotypes in f ( n =3, 3, 2, 3, 2 and 2 animals used per genotype, respectively). ( h ) Quantification of TUNEL staining ( n =6, 10, 4 and 4 sections per animal were scored, sections from 2, 3, 1 and 1 animals per genotype were used, respectively). ( i ) Misplacement of neural/stem cell progenitors (Sox2 positive) in Cep63 T/T and Cep63 T/T p53 −/− animals (scale bar, 50 μm). ( j ) Rescue of misplaced progenitors in Cep63 T/T p53 −/− animals compared with Cep63 T/T ( n =5, 3 and 3 animals per genotype, respectively). All graphics with error bars are presented as the average plus s.d. Asterisks denote statistical significance (* P value <0.05, ** P value <0.01 and *** P value<0.001) determined by the unpaired two-way Student’s t -test ( b , g , h , j ). Full size image To determine whether p53 activation was sufficient to drive NPC attrition in Cep63 T/T mice, we intercrossed them with p53 −/− animals. Strikingly, we observed a complete rescue of brain size in Cep63 T/T p53 −/− mutants ( Fig. 3e–g ). Consistent with these observations, terminal deoxynucleotidyl transferase dUTP nick end labeling (TUNEL) staining revealed increased numbers of apoptotic cells in E14.5 cortices of Cep63 T/T mice, which was rescued by loss of p53 ( Fig. 3h ). To determine whether the loss of p53 rescued the proliferating NPC population, we stained the cortex with antibodies for the NPC marker SOX2 and quantified cell number ( Fig. 3i,j ) [32] . In the Cep63 T/T cortex, we found a reduced total number of SOX2 positive cells but an increased percentage that were mislocalized ( Fig. 3j ). The reduction of NPC number in Cep63 T/T mice was rescued by p53 but the majority of the rescued NPCs were misplaced from the VZ (extra VZ), consistent with the loss of this misplaced progenitor population underlying the microcephaly phenotype ( Fig. 3i,j ). In response to DNA double-stranded breaks, the CHK2 and ATM kinases play important roles in mediating p53-dependent apoptosis [33] . However, in contrast to p53 deficiency, neither the loss of CHK2 nor ATM rescued the reduced brain size observed in Cep63 T/T animals ( Fig. 3f,g ). This suggested that chromosome breaks are unlikely to be a primary trigger for p53 activation and cellular attrition in vivo , consistent with the lack of extensive γH2AX staining ( Fig. 3c,d ). In addition, we have observed normal ATM/ATR-dependent DDR in MEFs and intact physiological repair in the immune system of Cep63 T/T mice ( Supplementary Fig. 2 ). Collectively, our data showed that CEP63 deficiency causes centrosomal defects that lead to mitotic errors and misplacement of NPCs, triggering p53-mediated cell death and microcephaly. Severe defects in testes development and male infertility While our assays failed to detect clear DDR defects in the brain ( Fig. 3c,d ) or other tissues ( Supplementary Fig. 2 ), we next examined fertility, as germline meiotic recombination is mediated by proteins largely distinct from those required for immune system development, and is often affected in genetic instability disorders [33] . We found that Cep63 T/T females were fertile and generated litter sizes comparable to those of WT animals ( Supplementary Fig. 3 ). However, histological examination found a reduction in the number of oocytes, even though follicles at all stages were present ( Supplementary Table 1 ). In contrast, despite copulation, no WT females were impregnated by Cep63 T/T males. We observed a progressive reduction in testis size in Cep63 T/T males, which was apparent in 10-day-old (p10) animals but more marked in 5.5-month-old (p165) animals ( Fig. 4a ), and was independent of p53, ATM or CHK2 ( Supplementary Fig. 4 ). Examination of 5-day-old (p5) Cep63 T/T animals revealed reduced cellularity but proportionally normal numbers of spermatagonia ( Fig. 4b ). In addition, we could occasionally identify polyploid spermatagonia in testes squash preparations, suggesting defective primordial germ cell expansion during development ( Fig. 4b ). Testes of p60 Cep63 T/T animals contained numbers of tubules comparable to WT, but tubule diameter and cellularity were reduced ( Fig. 4c,d and Supplementary Fig. 4 ), most likely due to increased cell death ( Fig. 4e,f ). Few spermatids were visible in Cep63 T/T testes sections, and rare elongated spermatids were identified in testes squash preparations, but all appeared morphologically abnormal, in some cases exhibiting defective DNA compaction as sperm tails stained with DAPI ( Fig. 4g ). Further, sperm counts from the dissected vas deferens showed that Cep63 T/T mice had no identifiable sperm, indicating that the rare Cep63 T/T spermatids did not leave the testes ( Fig. 4h ). These results suggested that CEP63 deficiency impairs spermatogenesis at multiple stages. 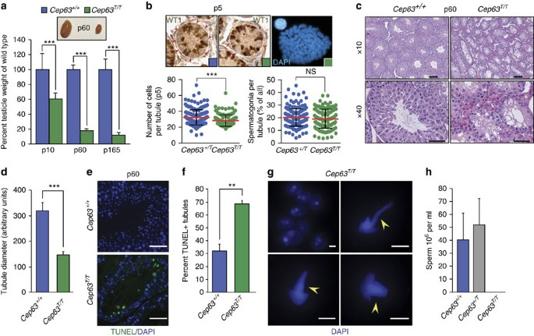Figure 4: Infertility and severe defects in testes development inCep63T/Tmice. (a) Comparison of testicle weight to WT littermates at p10, p60 and p165. Examples of dissected p60 testes are shown (n=4, 3, 8, 8, 2 and 4 animals, respectively). (b) Testes sections from p5 animals were stained with antibody against WT1 (upper panels) and WT1-negative cells (spermatagonia, red arrows) were scored and plotted (lower panels). Reduced cell numbers in p5 tubules (bottom left panel) but proportionally similar numbers of spermatagonia (bottom right panel) were observed (results are combined from fourCep63+/Tand threeCep63T/Tanimals. ForCep63+/Tn=201 andCep63T/Tn=143 tubules scored). Individual values are shown in a scatterplot with the average (red line) and s.d. (black lines) indicated. Tetraploidy was observed in some spermatagonia fromCep63T/Tanimals (upper right panel). (c) Haematoxylin and eosin staining of testes sections from p60 mice showing relative size and condition of tubules (scale bars, 100 μm in × 10 panels and 50 μm in × 40 panels). (d) Quantification of tubule size in the indicated genotypes (two animals per genotype,n=6 tubules per genotype measured). (e) Examples of TUNEL staining (scale bars, 50 μm). (f) Quantification of TUNEL-positive tubules (n=3 animals per genotype used, 279Cep63+/+and 266Cep63T/Ttubules scored). (g) Examples of aberrant spermatids fromCep63T/Ttestes squashes. DAPI-stained tails are indicated with yellow arrow heads (scale bars, 5 μm). (h) Sperm counts from mice of the indicated genotypes (n=4, 2 and 4 animals per genotype, respectively). All graphs with error bars are presented as the average plus s.d. Asterisks denote statistical significance (NS, not significant, **Pvalue <0.01 and ***Pvalue<0.001) determined by the unpaired two-way Student’st-test (a,d,f) or the unpaired two-way Wilcoxon rank-sum test (b). Figure 4: Infertility and severe defects in testes development in Cep63 T/T mice. ( a ) Comparison of testicle weight to WT littermates at p10, p60 and p165. Examples of dissected p60 testes are shown ( n =4, 3, 8, 8, 2 and 4 animals, respectively). ( b ) Testes sections from p5 animals were stained with antibody against WT1 (upper panels) and WT1-negative cells (spermatagonia, red arrows) were scored and plotted (lower panels). Reduced cell numbers in p5 tubules (bottom left panel) but proportionally similar numbers of spermatagonia (bottom right panel) were observed (results are combined from four Cep63 +/T and three Cep63 T/T animals. For Cep63 +/T n =201 and Cep63 T/T n =143 tubules scored). Individual values are shown in a scatterplot with the average (red line) and s.d. (black lines) indicated. Tetraploidy was observed in some spermatagonia from Cep63 T/T animals (upper right panel). ( c ) Haematoxylin and eosin staining of testes sections from p60 mice showing relative size and condition of tubules (scale bars, 100 μm in × 10 panels and 50 μm in × 40 panels). ( d ) Quantification of tubule size in the indicated genotypes (two animals per genotype, n =6 tubules per genotype measured). ( e ) Examples of TUNEL staining (scale bars, 50 μm). ( f ) Quantification of TUNEL-positive tubules ( n =3 animals per genotype used, 279 Cep63 +/+ and 266 Cep63 T/T tubules scored). ( g ) Examples of aberrant spermatids from Cep63 T/T testes squashes. DAPI-stained tails are indicated with yellow arrow heads (scale bars, 5 μm). ( h ) Sperm counts from mice of the indicated genotypes ( n =4, 2 and 4 animals per genotype, respectively). All graphs with error bars are presented as the average plus s.d. Asterisks denote statistical significance (NS, not significant, ** P value <0.01 and *** P value<0.001) determined by the unpaired two-way Student’s t -test ( a , d , f ) or the unpaired two-way Wilcoxon rank-sum test ( b ). Full size image CEP63 is required for male meiotic recombination As the position of TUNEL-positive cells in seminiferous tubules ( Fig. 4e ) was consistent with that of the meiotic population, we examined meiotic progression using markers for the lateral and central elements of the synaptonemal complex (SCP3 and SCP1, respectively). Compared with WT, Cep63 T/T mice showed increased leptotene and zygotene stage cells, similar numbers of pachytene cells but very few cells (4%) that progressed to diplotene ( Fig. 5a ). This suggested that defects in the early stages of meiotic prophase I delayed progression to later stages and/or there was progressive cell loss during prophase I. 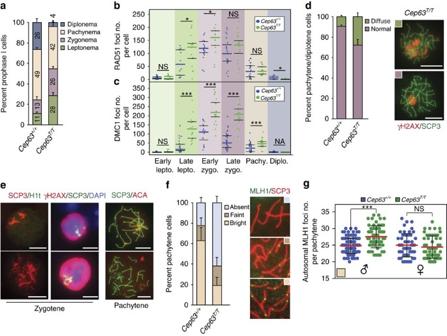Figure 5: Impaired meiotic progression inCep63T/Tmice. (a) Quantification of prophase I stages in meiotic cells of the indicated genotype based on co-staining of SCP1 and SCP3 (n=3 animals per genotype used, 289Cep63+/+and 301Cep63T/Tcells scored). Quantification of RAD51 (b) and DMC1 (c) foci in the indicated stages of prophase I (assessed by SCP3 staining) from the indicated genotypes (Cep63+/+n=112 and 157,Cep63T/Tn=122 and 108 cells scored, respectively). (d) Quantification of γH2AX staining patterns in pachytene and diplotene cells (n=3 animals per genotype used, 124Cep63+/+and 97Cep63T/Tcells scored), example spermatocyte spreads shown (scale bars, 10 μm). (e) Examples of aberrant SC structures observed in zygotene and pachytene spermatocytes fromCep63T/Tspreads (scale bars, 10 μm). (f) Quantification of crossover formation using MLH1 staining. Reduced numbers ofCep63T/Tpachytene cells have visible MLH1 foci (n=3 animals per genotype used, 84 and 59 cells scored, respectively). Examples of categories scored are shown in right panels. (g) Scoring of MLH1 foci in pachytene cells with visible MLH1 foci. In the low percentage ofCep63T/Tmales that have visible foci, there is a significant increase in foci number (n=101 and 135 cells scored). MLH1 foci in females is comparable regardless of genotype (Cep63+/+ or +/−n=2 (male)/2 (female) andCep63T/Tn=3 (male)/2 (female) animals). Individual values are shown in a scatterplot with the average (red line) and s.d. (black lines) indicated. All graphs with error bars are presented as the average plus s.d. Asterisks denote statistical significance (NS, not significant; NA, not applicable; *Pvalue <0.05 and ***Pvalue <0.001) determined by the unpaired two-way Wilcoxon rank-sum test (b,c,g). Diplo., diplotene; lepto., leptotene; pachy., pachytene; zygo., zygotene. Figure 5: Impaired meiotic progression in Cep63 T/T mice. ( a ) Quantification of prophase I stages in meiotic cells of the indicated genotype based on co-staining of SCP1 and SCP3 ( n =3 animals per genotype used, 289 Cep63 +/+ and 301 Cep63 T/T cells scored). Quantification of RAD51 ( b ) and DMC1 ( c ) foci in the indicated stages of prophase I (assessed by SCP3 staining) from the indicated genotypes ( Cep63 +/+ n =112 and 157, Cep63 T/T n =122 and 108 cells scored, respectively). ( d ) Quantification of γH2AX staining patterns in pachytene and diplotene cells ( n =3 animals per genotype used, 124 Cep63 +/+ and 97 Cep63 T/T cells scored), example spermatocyte spreads shown (scale bars, 10 μm). ( e ) Examples of aberrant SC structures observed in zygotene and pachytene spermatocytes from Cep63 T/T spreads (scale bars, 10 μm). ( f ) Quantification of crossover formation using MLH1 staining. Reduced numbers of Cep63 T/T pachytene cells have visible MLH1 foci ( n =3 animals per genotype used, 84 and 59 cells scored, respectively). Examples of categories scored are shown in right panels. ( g ) Scoring of MLH1 foci in pachytene cells with visible MLH1 foci. In the low percentage of Cep63 T/T males that have visible foci, there is a significant increase in foci number ( n =101 and 135 cells scored). MLH1 foci in females is comparable regardless of genotype ( Cep63 +/+ or +/− n =2 (male)/2 (female) and Cep63 T/T n =3 (male)/2 (female) animals). Individual values are shown in a scatterplot with the average (red line) and s.d. (black lines) indicated. All graphs with error bars are presented as the average plus s.d. Asterisks denote statistical significance (NS, not significant; NA, not applicable; * P value <0.05 and *** P value <0.001) determined by the unpaired two-way Wilcoxon rank-sum test ( b , c , g ). Diplo., diplotene; lepto., leptotene; pachy., pachytene; zygo., zygotene. Full size image The efficient generation of DNA double-strand breaks (DSBs) in leptotene and their subsequent repair is required for timely homologue pairing, synapsis and meiotic prophase progression [34] , [35] . We examined the number of DSBs generated during prophase I by counting the number of foci of the repair proteins RAD51 and DMC1. Increased numbers of RAD51 and DMC1 foci were observed from leptotene to zygotene in Cep63 T/T mice compared with WT ( Fig. 5b,c ), suggesting that formation of DSBs was not defective, but their resolution potentially was. In Cep63 T/T cells that progressed to pachytene, foci were largely resolved to similar levels as in WT. However, many pachytene and diplotene cells exhibited diffuse γH2AX staining that was not confined to the sex–body, consistent with delayed repair ( Fig. 5d ). We also identified numerous abnormal or apoptotic cells with zygotene- and pachytene-like SC patterns (H1t negative, a marker of late pachytene) that were absent in controls ( Fig. 5e ). These included apparent SC entanglements and chromosome fusions, as well as ring γH2AX staining, indicative of programmed cell death ( Fig. 5e ). We next examined crossover formation, one of the outcomes of meiotic recombination, using MLH1 as a marker. In contrast to WT, the majority of pachytene cells from male Cep63 T/T mice lacked detectable MLH1 foci ( Fig. 5f ), indicating that they did not progress past early pachytene, an observation corroborated by H1t staining ( Supplementary Fig. 4 ). In cases where MLH1 foci were present, higher numbers of crossovers per autosome ( Fig. 5g ) and longer SCs were detectable ( Supplementary Fig. 4 ), reinforcing a role for CEP63 in the completion of male meiotic recombination. In contrast, comparable numbers of MLH1 foci were observed in WT and Cep63 T/T females, supporting a sex-specific role for CEP63 during meiotic prophase I progression ( Fig. 5g ). Thus, the loss of CEP63 led to male-specific meiotic recombination defects, cell death and infertility. Impaired centriole duplication in CEP63-deficient cells As the severe recombination defect we observed was unexpected, given that we have not detected sensitivity to DNA damage or nuclear localization of CEP63 or CEP152 in other tissues, we examined their localization throughout prophase I using SCP3 as a marker. Regardless of the stage, CEP63 or CEP152 localization was restricted to centrosomes, identified by staining with PCNT ( Fig. 6a ). Consistent with what we observed in all other cell types and tissues we have examined, centrosomal CEP63 and CEP152 were not detected in prophase I spermatocytes in the testes of Cep63 T/T mice ( Fig. 6a ). 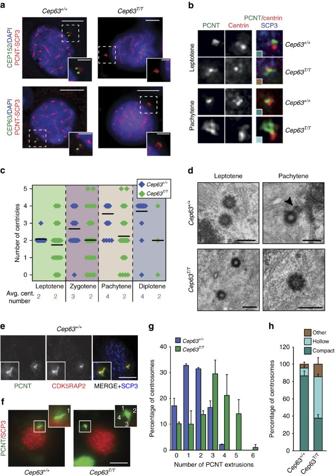Figure 6: Centriole duplication failure during meiotic prophase I inCep63T/Tmice. (a) CEP152 and CEP63 are detectable at centrosomes, marked by PCNT, in the SCP3-staged prophase I cells of WT (left panels) but notCep63T/T(right panels) (scale bars, 5 μm (left) and 2 μm (right)). (b) Example images of centriole configurations detected by immunofluorescence microscopy in spermatocytes at the indicated stage and of the indicated genotype. The colours of the insets correspond to the colours used for the graph inh. (c) Quantification of centriole numbers in prophase I spermatocytes at the indicated stage and of the indicated genotype. Example images are shown inband inSupplementary Fig. 5. Average (Avg.) centriole (cent.) number per stage is indicated (black line) and the value rounded to a whole number shown numerically below (three animals per genotype used,Cep63+/+n=121,Cep63T/Tn=130 cells scored). (d) TEM analysis of centriole configurations in WT andCep63T/Tspermatocytes at the indicated stages. The arrowhead points to a daughter centriole growing from the wall of the mother (scale bars, 400 nm). (e) Co-distribution of the two PCM markers PCNT and CDK5RAP2 in squashes of WT spermatocytes. SCP3 staining was used for staging. (f) Examples of PCM extrusion patterns detected by PCNT staining in WT andCep63T/Tspermatocyte squashes. SCP3 staining was used for staging. The insets show magnifications of the PCM region, with extrusions labelled by numbers (scale bar, 5 μm). (g) Quantification of centrosome extrusions (PCNT staining) in spermatocytes of the indicated genotypes (n=2 animals per genotype used, 92Cep63+/+and 87Cep63T/Tcells scored). (h) Quantification of PCM distribution (PCNT staining) patterns in spermatocytes from WT andCep63T/Tmice (n=3 animals per genotype used, 121Cep63+/+and 130Cep63T/Tcells scored). Additional PCM marker analysis is included inSupplementary Fig. 6. All graphs with error bars are presented as the average plus s.d. Figure 6: Centriole duplication failure during meiotic prophase I in Cep63 T/T mice. ( a ) CEP152 and CEP63 are detectable at centrosomes, marked by PCNT, in the SCP3-staged prophase I cells of WT (left panels) but not Cep63 T/T (right panels) (scale bars, 5 μm (left) and 2 μm (right)). ( b ) Example images of centriole configurations detected by immunofluorescence microscopy in spermatocytes at the indicated stage and of the indicated genotype. The colours of the insets correspond to the colours used for the graph in h . ( c ) Quantification of centriole numbers in prophase I spermatocytes at the indicated stage and of the indicated genotype. Example images are shown in b and in Supplementary Fig. 5 . Average (Avg.) centriole (cent.) number per stage is indicated (black line) and the value rounded to a whole number shown numerically below (three animals per genotype used, Cep63 +/+ n =121, Cep63 T/T n =130 cells scored). ( d ) TEM analysis of centriole configurations in WT and Cep63 T/T spermatocytes at the indicated stages. The arrowhead points to a daughter centriole growing from the wall of the mother (scale bars, 400 nm). ( e ) Co-distribution of the two PCM markers PCNT and CDK5RAP2 in squashes of WT spermatocytes. SCP3 staining was used for staging. ( f ) Examples of PCM extrusion patterns detected by PCNT staining in WT and Cep63 T/T spermatocyte squashes. SCP3 staining was used for staging. The insets show magnifications of the PCM region, with extrusions labelled by numbers (scale bar, 5 μm). ( g ) Quantification of centrosome extrusions (PCNT staining) in spermatocytes of the indicated genotypes ( n =2 animals per genotype used, 92 Cep63 +/+ and 87 Cep63 T/T cells scored). ( h ) Quantification of PCM distribution (PCNT staining) patterns in spermatocytes from WT and Cep63 T/T mice ( n =3 animals per genotype used, 121 Cep63 +/+ and 130 Cep63 T/T cells scored). Additional PCM marker analysis is included in Supplementary Fig. 6 . All graphs with error bars are presented as the average plus s.d. Full size image During meiotic prophase, membrane spanning Linker of Nucleoskeleton and Cytoskeleton (LINC) complexes containing SUN and KASH domain proteins tether chromosomes to the inner nuclear envelope and mediate interactions with the microtubule cytoskeleton at the cytoplasmic side [36] . This linkage drives chromosome movements and facilitates correct meiotic homologue pairing and recombination [37] , [38] , [39] , [40] . We therefore speculated that recombination failure in Cep63 T/T males could be due to aberrant centrosomes. To address this, we first characterized centriole duplication in WT spermatocytes since, to our knowledge, the unperturbed centrosome configuration in mouse prophase I spermatocytes had not been reported previously. By staining with antibodies against PCNT and centrin 3 to label centrosomes and centrioles, and SCP3 antibodies for meiotic staging, we found that early prophase I spermatocytes presented a single centrosome (single PCNT-positive foci) with unduplicated centrioles (two small centrin-positive dots adjacent to the larger PCNT foci) ( Fig. 6b,c and Supplementary Fig. 5 ). At later stages, centriole numbers increased, and only by pachytene/diplotene, centriole duplication was completed (four centrin dots) ( Fig. 6c and Supplementary Fig. 5 ). Separation of duplicated centrosomes occurred only at the end of prophase I or early in prometaphase I ( Supplementary Fig. 5 ). Consistent with this, CEP63 and CEP152, which are associated with the proximal end of mother centrioles [5] , localized as two foci that remained paired from leptotene through pachytene ( Fig. 6a ). Interestingly, staining with anti-NEDD1 or anti-γ-tubulin antibodies, which detect the microtubule nucleating γ-tubulin ring complex, was relatively dim and restricted to the centrioles throughout prophase I ( Supplementary Fig. 5 ). Together, the data suggest that contrary to the situation in most somatic cells, centrosome duplication and separation in mouse spermatocytes are delayed, such that duplication is initiated in early prophase I and duplicated centrosomes are not separated before the end of prophase I. To validate these findings, we used transmission electron microscopy (TEM). Consistent with the immunofluorescence results, WT spermatocytes in leptotene always contained a single centrosome with unduplicated centrioles ( Fig. 6d ). Only at zygotene/pachytene could short daughter centrioles growing from the wall of mother centrioles be observed ( Fig. 6d ). By metaphase I, mothers and elongated daughters that appeared disengaged were present at spindle poles ( Supplementary Fig. 5 ). This was consistent with previous work that reported essentially the same pattern of delayed centriole duplication and centrosome separation in hyrax and squirrel spermatocytes [41] . Next, we analysed centrosomes in Cep63 T/T spermatocytes. In contrast to WT cells, many Cep63 T/T cells had only one or no detectable centriole at leptotene, and most existing centrioles failed to duplicate during prophase I. As a result, by pachytene/diplotene, Cep63 T/T cells contained on average only two centrioles, whereas WT cells contained four ( Fig. 6c and Supplementary Fig. 5 ). TEM analysis confirmed the presence of only one or two single centrioles in leptotene ( Fig. 6d ). Interestingly, in cells with two centrioles, these appeared to be slightly further apart than in WT cells ( Fig. 6d ). Strikingly, we never observed growing or fully grown daughter centrioles at later stages. Despite the duplication defect, the existing centrioles in Cep63 T/T cells appeared to be of normal size and structure, consistent with previous results in chicken DT40 cells lacking CEP63 ( Supplementary Fig. 6 ) [5] . Apart from impairing centriole duplication CEP63 deficiency also seemed to affect centrosome integrity. PCNT staining of WT centrosomes revealed an irregularly shaped but compact pericentriolar material (PCM), which in most cells had one or two extrusions ( Fig. 6e–g ). The identity and distribution of the PCM was confirmed by two independent markers, CDK5RAP2 and PCNT, which largely colocalized ( Fig. 6e ). Compared with WT cells, the PCM of centrosomes in Cep63 T/T spermatocytes appeared less compact, with a less intensely stained central region (‘hollow’) and an increase in extrusion number ( Fig. 6b,e–h ). However, total levels of PCNT at centrosomes were similar in WT and Cep63 T/T spermatocytes ( Supplementary Fig. 6 ). Very similar PCM perturbations in Cep63 T/T cells were revealed by staining with CDK5RAP2 antibodies ( Supplementary Fig. 6 ). Together, these data indicated that in spermatocytes, CEP63 was crucial for centriole duplication during meiotic prophase I, and that even though centriolar ultrastructure appeared normal, most centrosomes lacking CEP63 displayed abnormal PCM organization. Telomere clustering defects in CEP63-deficient cells As a direct role for CEP63/CEP152 in meiotic recombination seemed unlikely given the lack of detectable nuclear localization, we asked whether aberrant centrosomes in Cep63 T/T cells impair chromosome movements required for recombination. Such a defect could be caused by loss of chromosome attachment to the nuclear envelope or lack of tethering to the microtubule cytoskeleton by LINC complexes [40] , [42] , [43] . In Cep63 T/T spermatocytes, SUN1, the telomeric SUN domain protein that mediates attachment of chromosomes to the inner nuclear envelope, was localized to telomeres, and the distribution of TRF1 (telomeric marker) was consistent with nuclear envelope localization ( Fig. 7a ), suggesting that chromosome attachment was intact. We next analysed the outcome of chromosome tethering to the microtubule cytoskeleton by quantifying ‘bouquets’, a leptotene/zygotene chromosome configuration that arises from transient clustering of chromosome termini [39] . Staining with ACA antibodies to label the centromeric ends of mouse acrocentric chromosomes and SCP3 antibodies for staging revealed a significant reduction in telomere clustering in Cep63 T/T spermatocytes of juvenile mice compared with WT ( Fig. 7b,c ). Together, our data suggests that in spermatocytes, CEP63 loss triggers cell death independently of p53, ATM or CHK2, primarily as a consequence of defective meiotic recombination, rather than mitotic spindle errors. Considering that CEP63 and CEP152 are physically separated from the chromosomes and can only be detected at centrosomes throughout prophase I ( Fig. 6a ), and that PCM organization is impaired in CEP63-deficient cells ( Fig. 6e–h ), we propose that these errors are likely caused by aberrant centrosomes that impair normal intranuclear chromosome movements ( Fig. 7d ). 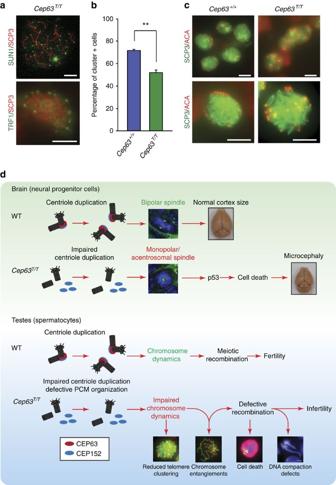Figure 7: Reduced telomere clustering inCep63T/Tmice. (a) Telomeric attachment in spermatocytes visualized by staining with SUN1 (top picture—pachytene spread, scale bar, 10 μm) or TRF1 (lower picture—equatorial plane from pachytene squash, scale bar, 5 μm). (b) Quantification of cells with clustered telomeres, indicative of bouquet formation, in p10 spermatocytes of the indicated genotype (Cep63+/+n=4 andCep63T/Tn=5 animals per genotype used, 274 and 407 cells scored, respectively). Graph with error bars shows the average plus s.d. Asterisks denote statistical significance (**Pvalue<0.01) determined by an unpaired two-way Student’st-test. (c) Representative squash images from cells of the indicated genotype staining with ACA (centromere/telomere) and SCP3 (SC), scale bar, 5 μm. (d) Model of CEP63 function in normal brain and testes development. See text for description. Figure 7: Reduced telomere clustering in Cep63 T/T mice. ( a ) Telomeric attachment in spermatocytes visualized by staining with SUN1 (top picture—pachytene spread, scale bar, 10 μm) or TRF1 (lower picture—equatorial plane from pachytene squash, scale bar, 5 μm). ( b ) Quantification of cells with clustered telomeres, indicative of bouquet formation, in p10 spermatocytes of the indicated genotype ( Cep63 +/+ n =4 and Cep63 T/T n =5 animals per genotype used, 274 and 407 cells scored, respectively). Graph with error bars shows the average plus s.d. Asterisks denote statistical significance (** P value<0.01) determined by an unpaired two-way Student’s t -test. ( c ) Representative squash images from cells of the indicated genotype staining with ACA (centromere/telomere) and SCP3 (SC), scale bar, 5 μm. ( d ) Model of CEP63 function in normal brain and testes development. See text for description. Full size image Cep63 -deficient mice recapitulate two key aspects of human Seckel syndrome associated with CEP63 mutations (SCKL6): growth retardation and microcephaly [5] . Our analysis suggests that the aetiology of microcephaly in Cep63 T/T animals is partially distinct from that reported for Atr or Mcph1 . Atr deficiency causes more severe facial dysmorphia and runting than either Mcph1 or Cep63 deficiency [24] , [44] . In addition, deletion of p53 in Atr -deficient animals exacerbates the neurodevelopmental phenotypes, whereas deletion of p53 in Cep63 T/T mice rescued microcephaly ( Fig. 3e–g ). Rescue of microcephaly following p53 deletion has also been reported in other models with more severe centriole loss [25] . Microcephaly in Mcph1 -deficient mice has been linked to abrogated CHK1 recruitment to centrosomes and premature CDK1 activation that compromises the timing of division modes and self-renewal capacity of NPCs, resulting in their premature decline [27] . While we observed reduced neurosphere forming capacity of NPCs from Cep63 T/T embryos, we did not observe a progressive decline, as was reported in Mcph1 mutants, suggesting that self-renewal defects are likely not the major cause of NPC depletion in Cep63 T/T mice ( Supplementary Fig. 7 ). In addition, previous work has implicated CEP63 in CDK1 recruitment to centrosomes, arguing against a mechanism of premature centrosomal CDK1 activation [27] , [45] . However, this issue will require further investigation since some of the CDK1 antibodies used for cytology crossreact with CEP152, that we, and others, have shown is dependent on CEP63 for centrosomal recruitment ( Fig. 2a and 6a ) [5] , [22] , [46] , [47] . We propose that defective CEP63/CEP152-dependent centriole duplication in Cep63 T/T mice leads to mitotic spindle defects in NPCs, including monopolar spindles and acentriolar spindle poles ( Fig. 7d ), as well as detachment and mislocalization of NPCs. This phenotype is very similar to what has been reported recently in mice lacking the essential centriole biogenesis factor SAS4 (ref. 25 ) and is consistent with the previous proposition that centriole duplication defects in NPCs may be a major cause of human primary microcephaly [48] . Mitotic failure and subsequent G1 entry could result in polyploidy, which we have clearly observed in several Cep63 T/T cell types ( Fig. 4b and Supplementary Fig. 2 ) and has also been reported in other systems [45] . However, an in-depth fluorescence in situ hybridization analysis in the developing cortex of SAS4-depleted animals, which have an even more marked centriole loss phenotype than Cep63 T/T mice, was unable to detect aneuploid cells, suggesting that stringent control mechanisms exist in the murine brain to prevent the accumulation of aneuploid cells [5] , [45] . We believe that available data support the idea that acentrosomal spindles and resulting mitotic spindle defects lead to mitotic delays that trigger p53-dependent cell death and promote microcephaly in Cep63 T/T animals [26] , [49] . Such a mechanism would also be consistent with the inability of Chk2 or Atm mutations to rescue the phenotype ( Fig. 3f,g ), the lack of extensive γH2AX staining ( Fig. 3c ), and the grossly normal DDR we have observed in cultured fibroblasts and during the immunological development of Cep63 T/T mice ( Supplementary Fig. 2 ). We have not obtained any evidence for defects in ATM/ATR-related signalling in Cep63 T/T mice, and the ATM/ATR-dependent phosphorylation site identified in frog and chicken CEP63 is not conserved in the mammalian protein. However, as additional ATM/ATR consensus phosphorylation sites [50] exist in CEP63, it remains possible that CEP63 is a target of ATM/ATR or other damage-induced modifications that affect its function after DNA damage. It also remains possible that the CEP63 paralogue, Deup1 , provides some compensation, although we did not see evidence of increased Deup1 mRNA levels in the brain ( Fig. 1e ) [51] . As CEP63 has been described to interact with the UVRAG protein that influences DNA repair and autophagy, we cannot exclude that CEP63 has a role in the damage responses in tissues that we have not investigated or affects the DDR in a more subtle manner than can be detected by our assays [52] . Several mouse mutants in MCPH and Seckel genes exhibit both male and female subfertility or infertility [15] , [53] . To our knowledge, this is the first example of male-specific infertility associated with these disorders, but as only three female SCKL6 patients have been identified to date [5] , we cannot confirm that this is the case in humans. The severity of the phenotype was surprising given the apparently normal DNA repair programs in the immune system ( Supplementary Fig. 2 ), as well as the fertility and normal recombination observed in Cep63 T/T females ( Fig. 5g , Supplementary Fig. 3 and Supplementary Table 1 ). Centrioles can be detected in oocytes by TEM up to the pachytene stage [54] , [55] , but whether these represent bona fide centrosomes is unclear. We speculate that distinct requirements for the organization and function of the centrosome during meiotic prophase in males and females may explain the marked sex specificity we observe. Meiotic recombination is the only DNA repair defect we have observed thus far in Cep63 T/T mice or cell cultures. During prophase I, chromosomes are physically separated from the centrosome by the nuclear envelope, and, in contrast to MCPH1 or ATR, we have seen no evidence for CEP63 nuclear translocation, although the limitations of the available immunoreagents preclude the definitive exclusion of this possibility ( Fig. 6a ) [15] , [22] , [56] . The major difference between homologous recombination in mitotic and meiotic cells is the use of the homologue, rather than the sister chromatid, as a template. As homologous chromosomes may be further apart than sister chromatids, global chromosome movements are likely to be required to facilitate timely homologue location and pairing. In addition, rapid chromosome movements have been proposed to dissociate non-homologous chromosome interactions [39] , [57] , [58] , [59] , [60] . The centrosome is the major microtubule-organizing centre, and its composition and functions are defective in the absence of CEP63, potentially compromising the microtubule network and leading to impaired chromosome dynamics. This would be consistent with the fact that we have observed decreased telomere clustering, meiotic DNA repair defects and aberrant chromosome entanglements and fusions in CEP63-deficient mice ( Fig. 7d ). While chromosome positioning LINC complexes have also been implicated in neuronal pathology and infertility [20] , defects in the interactions between the centrosome, microtubules and LINC complexes in Cep63 -deficient animals could also play a role in other aspects of development. In summary, our study has identified critical roles for CEP63 during brain development and suggests that increased p53-dependent cell death during embryogenesis could be the sole cause of microcephaly in some forms of Seckel syndrome and MCPH in human patients. In addition, it indicates that similar pathways are activated during neural development in response to acentrosomal and multicentrosomal spindle configurations [26] , [28] . Future studies will be required to address the precise trigger(s) for p53 activation and to determine how generally this genetic dependency extends to other disorders resulting from centrosome defects. In addition, we have also uncovered an unexpected role for CEP63 in meiotic recombination, establishing the crosstalk between centrosome and recombination machinery as crucial for the fidelity of male gamete generation. Generation and husbandry of mice The generation of Cep63 gene-trapped mice was described previously [22] . Mice lacking p53 were purchased from Jackson Laboratories, Chk2 -deficient mice were obtained from Tak Mak [61] and Atm-deficient mice were obtained from Anthony Winshaw-Boris [62] . All animals were maintained on a mixed 129/SvEv-C57BL/6 background in strict accordance with the European Community (86/609/EEC) guidelines at the animal facilities in the Barcelona Science Park (PCB). Protocols were approved by the Animal Care and Use Committee of the PCB (IACUC; CEEA-PCB) in accordance with applicable legislation (Law 5/1995/GC; Order 214/1997/GC; Law 1201/2005/SG). All efforts were made to minimize use and suffering. Real-time quantitative PCR Dissected tissue or primary MEFs were collected on ice, washed in PBS and frozen. Tissues were disrupted in lysis buffer by zirconium beads in a mechanical tissue disruptor (Precellys 24, Bertin Technologies). RNA was isolated according to manufacturer recommendations (PureLink RNA mini kit, Ambion). An amount of 2 μg of RNA was used in a reverse transcriptase reaction using a high-capacity RNA-to-cDNA kit (Applied Biosystems). Amplification of the cDNA was done with TaqMan master mix and specific probes for Cep63, Anapc13, Plk4, Cep152 and Deup1. Probes for B2m and ACTB were used as housekeeping controls. Reactions were run on a 7900HT thermocycler (Applied Biosystems) and data were plotted using SDS2.3 software. The 2 −ΔΔCT method was used for the analysis of the amplification products. Sperm counts To determine sperm counts, cauda epididymis was dissected from 8- to 10-week-old mice, cut with scissors in five places and incubated in 1 ml of warm PBS at 37 °C for 10 min to let the sperm exit the tissue. After the incubation, sperm suspension was diluted 1:10 and manually counted under the microscope on the Neubauer glass slide counter. Meiotic spreads Testes from 8- to 10-week-old mice (unless stated otherwise) were dissected, tunica was removed and tubules containing germ cells were disaggregated using a razor blade followed by passage through a p1000 tip in 1 ml of media (Dulbecco’s modified Eagle medium supplemented with protease inhibitor cocktail, Roche 11873580001). The suspension was transferred to 5 ml of media and incubated for 5 min to precipitate larger pieces. Supernatant was distributed into 1 ml aliquots and centrifuged for 5 min at 7,500 r.p.m. The pellet was suspended in 40 μl of hypotonic buffer containing 0.1 M sucrose supplemented with protease inhibitors and 20 μl of cell suspension was added to 70 μl of fixing solution (1% paraformaldehyde (PFA) with 0.1% Triton X-100) on the glass slide that was incubated in a humidified incubation chamber. After 2 h, slides were rinsed with Ilfotol wetting agent (1:250 in water, Ilford) and processed immediately for immunofluorescence or stored at −80 °C for later use. Meiotic squashes Spermatocyte squashes were performed as previously described [63] , [64] . In brief, tubules from 10 days or 8–10-week-old mice (unless stated otherwise) were placed directly in fixative solution (2% formaldehyde, 0.05% Triton X-100 in PBS) for 10 min. To release spermatocytes from tubules, a small aliquot of the tubules was minced with tweezers on a glass slide pre-treated with poly- L lysine. Cells were covered with a coverslip and gently squashed by applying pressure with the thumb. The slide was snap-frozen in liquid nitrogen, the coverslip was removed and the slide was immediately processed for immunofluorescence. Alternatively, tubules were minced without fixation, squashed and frozen in liquid nitrogen. After removal of the coverslip, slides were fixed in ice-cold 95% ethanol for 10min followed by 4% formaldehyde for 7min (the latter protocol improves centrosome morphology). Immunofluorescence analysis Slides with spermatocytes were washed in blocking solution (1% BSA and 0.05% Tween-20 in PBS) for 30 min and then incubated with primary antibody overnight in a humidified chamber at 4 °C. Slides were washed multiple times in blocking solution and incubated with complementary Alexa Fluor-conjugated secondary antibody for 2 h at room temperature (RT). Slides were extensively washed with blocking solution, and in the last washing step DAPI was used as a counter stain (unless stated otherwise). Slides were then mounted using Prolong Gold antifade reagent (Life Technologies). For double-antigen staining, two primary antibodies of different origin were combined together in an overnight incubation. For triple-antigen staining, two primary antibodies of different origin were combined together in the first overnight incubation, then washed and incubated with complementary secondary antibodies. Third-antigen staining (mouse SCP3 in squashes, mouse γH2Ax in spreads) was incubated overnight and then visualized with Alexa Fluor 350-conjugated anti-mouse secondary antibody (Life Technologies). Immunohistochemistry Freshly dissected testes and ovaries of the indicated age were fixed in Bouin’s solution (Electron Microscopy Sciences) or in 10% neutral buffered formalin (5 days old testes) and embedded in paraffin using standard procedures. Sections were cut at 5 μm thickness and stained with haematoxylin and eosin (testes) or haematoxylin and Periodic acid/Schiff reagent (Sigma-Aldrich, testes and ovaries). Five-day-old testes were immunolabelled with WT1 antibody (Novus Biologicals) and counterstained with haematoxylin. P60 brains were dissected from animals and fixed overnight in 10% neutral buffered formalin (Sigma), embedded in paraffin using standard procedures and stained with haematoxylin and eosin. For brain cryosections, E14.5 mouse heads were fixed with 4% PFA for 48 h, cryoprotected in 30% sucrose and frozen in optimal cutting temperature (OCT) compound at -80°C. P2 animals were anaesthetized with ice and perfused intracardially with PBS followed by 4% PFA. Brains were removed, post fixed with 4% PFA overnight, cryoprotected in 30% sucrose and frozen in OCT at −80 °C. Cryosections were cut at 10 μm thickness and fixed to frosted glass slides by incubation for 20 min in ice-cold acetone at −20 °C. Slides were then washed several times in PBS followed with washing in PBS-T (0.3% Triton X-100 in PBS) and blocked with 5% goat serum in PBS-T for 60 min. Slides were incubated overnight at 4 °C with primary antibody, next day washed several times in PBS-T and stained with Alexa Fluor-conjugated complementary secondary antibody for 60 min at RT. After final washing, DNA was counterstained with Hoechst 33342. For SOX2 and TBR2 staining, an antigen retrieval procedure was performed before the blocking step by incubating tissue sections in citrate-based buffer for 5 min in a microwave pressure cooker at 70% power. For TUNEL staining, Bouin’s solution-fixed paraffin-embedded sections of 8–10-week-old mice testes or cryosections of 4% PFA-fixed mouse embryonic brains were labelled with In Situ Cell Death Detection Kit (TUNEL) according to the manufacturer’s instructions (Roche, 11684795910). For colorimetric visualization, sections were incubated with cleaved caspase-3 antibody overnight at RT after quenching endogenous peroxidase using 0.6% H 2 O 2 (vol/vol) in methanol. Slides were washed with PBS three times, followed by incubation with biotinylated secondary antibody and avidin–biotin complex (Vectastain Elite kit, Vector Labs). Immunoreactive signals were visualized with the VIP substrate kit (Vector Labs) using the manufacturer's protocol. Sections were counterstained with 0.1% methyl green (wt/vol), dehydrated and mounted in DPX (Fluka). Antibodies Primary antibodies are listed in Supplementary Table 2 . Secondary antibodies used were as follows: fluorescein isothiocyanate- and Cy3-conjugated secondary antibodies (Jackson Immunologicals), Alexa Fluor 350-, 488- and 568-conjugated goat anti-mouse, Alexa Fluor 488- and 568-conjugated goat anti-rabbit, Alexa Fluor 488-conjugated goat anti-guinea pig and Alexa Fluor 568-conjugated anti-human antibodies (Life Technologies). Microscopy Brain histological sections were imaged with a macroscope (Olympus MVX10) and neocortical thickness was measured in comparative sections from the pia to the white matter. At p2, cortical thickness was measured in the motor, somatosensory and visual cortex (2.31, 3.75 and 4.23 mm, respectively, according to ref. 65 ) and at p60 in motor and visual cortex (Bregma: 1.42 and -2.70, respectively). Fluorescent images were acquired with an Orca AG camera (Hamamatsu) mounted on a Leica DMI6000B microscope equipped with 1.4 numerical aperture × 63 and × 100 oil immersion objectives. AF6000 software (Leica) was used for image acquisition and deconvolution of z-stack images (distance between z-slices was 0.2 μm). Coronal/sagittal serial brain sections from embryos at E14.5 from multiple animals per genotype were analysed in each experiment (details in figure legends). For cell counts in the cortex, all cells from the ventricular surface to the pial surface were counted and normalized with the area selected (mm 2 ). Additional image processing and maximum intensity z -projections were done in ImageJ software. Mitotic figure classification was done using apical mitosis within cortical sections imaged with a Leica TCS SP5 laser scanning spectral confocal microscope set-up on a Leica DMI600 inverted microscope. Confocal z-stacks were acquired with 0.2 μm of step size and using laser parameters that minimized the presence of saturated pixels. γ-Tubulin distribution in mitotic centrosomes was calculated assigning centrosomes to the ‘2 bright poles’ category when both γ-tubulin signals fell within the 40–60% of distribution of their bright/dim ratio, and ‘1 dim or absent pole’ category if one of the γ-tubulin signals fell within a 60–100% distribution of bright/dim ratio. Transmission electron microscopy Testes of mature mice were dissected and fixed for transmission EM analysis as previously described [66] . Briefly, testes were pre-fixed in cacodylate-buffered glutaraldehyde and post fixed in buffered OsO 4 followed by Renlam M-1 resin (Serva, Heidelberg, Germany). Ultrathin sections were analysed in a Tecnai12 BioTwin transmission EM (FEI, Eindhoven, NL) and imaged with a CCD camera (SIS MegaView3, Surface Imaging Systems, Herzogenrath, Germany) and the Analysis Imaging Interface. Contrast and brightness of images were further adjusted using Adobe Photoshop CS. Statistics All graphics with error bars are presented as average+s.d. (except in Fig. 6c where only average bar is shown and Figs 1a,b and 5b,c where median with first and third quartile of the box plot is shown. To determine statistical significance between samples, unpaired two-way Wilcoxon rank-sum test was used on samples with eight or more read-outs ( Figs 1b , 4b and 5b,c,g ), whereas in cases with <8 read-outs, unpaired two-way Student’s t -test was used ( Figs 1a,g and 2d,h , Figs 3b,d,g,h,j and 4a,d,f , and Fig. 7b ). Log-rank test was used for Kaplan–Meier comparison ( Fig. 1h ). Statistical calculations and generation of graphics were performed in Excel, R console, GraphPad Prism or Mstat (NS, nonsignificant; * P <0.05, ** P <0.01 and *** P <0.001). How to cite this article: Marjanović, M. et al. CEP63 deficiency promotes p53-dependent microcephaly and reveals a role for the centrosome in meiotic recombination. Nat. Commun. 6:7676 doi: 10.1038/ncomms8676 (2015).